Arabidopsis florigen FT binds to diurnally oscillating phospholipids that accelerate flowering Arabidopsis FT protein is a component of florigen, which transmits photoperiodic flowering signals from leaf companion cells to the shoot apex. Here, we show that FT specifically binds phosphatidylcholine (PC) in vitro . A transgenic approach to increase PC levels in vivo in the shoot meristem accelerates flowering whereas reduced PC levels delay flowering, demonstrating that PC levels are correlated with flowering time. The early flowering is related to FT activity, because expression of FT-effector genes is increased in these plants. Simultaneous increase of FT and PC in the shoot apical meristem further stimulates flowering, whereas a loss of FT function leads to an attenuation of the effect of increased PC. Specific molecular species of PC oscillate diurnally, and night-dominant species are not the preferred ligands of FT. Elevating night-dominant species during the day delays flowering. We suggest that FT binds to diurnally changing molecular species of PC to promote flowering. In many plant species, the time of flowering is largely regulated by day length or photoperiod. The long-day (LD) plant Arabidopsis thaliana perceives day length in leaves, where CONSTANS ( CO ) integrates circadian rhythm and light signal input to induce transcription of its major target gene, FLOWERING LOCUS T ( FT ) [1] . FT is a systemic inducer of flowering that is expressed in the companion cells of the phloem and exported to the phloem sieve elements from where it is transported to the shoot apex [2] , [3] , [4] . There are at least two critical steps in florigen signalling, export from companion cells to the sieve element and activation of its effector genes at the shoot apex that trigger subsequent flower development. FT protein expressed but immobilized in the companion cells is not able to promote flowering unless it is released to the phloem [4] . Indeed, FT-INTERACTING PROTEIN1 (FTIP1) is an essential ER-localized protein that interacts with FT and assists its transport from the phloem companion cells to the sieve elements [5] . The FT protein interacts with the bZIP transcription factor FD, which is expressed in the shoot apex and induces the expression of APETALA1 ( AP1 ) and SUPPRESSOR OF OVEREXPRESSION OF CONSTANS1 ( SOC1 ) to initiate flower development [6] , [7] , [8] . A rice paralog of FT, Hd3a, was shown to interact with the 14-3-3 protein GF14c at the shoot apex forming a bridge with a bZIP transcription factor related to FD [9] . This tripartite complex was named the florigen activation complex (FAC) [9] . Interestingly, crystallographic analysis of Hd3a as well as FT revealed a putative ligand-binding pocket in addition to the GF14c binding site, suggesting that another, as yet unidentified molecule binds to FT [9] , [10] . FT has long been recognized to be a homologue of phosphatidylethanolamine (PE)-binding protein (PEBP) from mammalian cells which shows affinity to PE [11] . Later, this PEBP was found to act as a Raf kinase inhibitor protein (RKIP), executing an inhibitory effect on the Raf kinase signalling cascade [12] . Although multiple lines of evidence show that mammalian PEBP/RKIP binds to different phospholipids, its physiological roles in vivo are still poorly understood. Therefore, the sequence similarity of FT with PEBP/RKIP suggests that phospholipids might represent novel binding partners of FT to modulate its function. Here, we show that in vitro FT specifically binds the phospholipid phosphatidylcholine (PC). A transgenic approach to increase PC levels in vivo in the shoot apical meristem accelerates flowering whereas reduced PC levels delay flowering, demonstrating that PC levels are correlated with flowering time. The early flowering is related to FT activity, because expression of two FT-effector genes, SOC1 and AP1 , is increased in these plants. Simultaneous increase of FT and PC in the shoot apical meristem further stimulates flowering, whereas a loss of FT function leads to an attenuation of the effect of increased PC. Specific molecular species of PC oscillates diurnally, and night-dominant species are not the preferred ligands of FT. Elevating night-dominant species of PC during the day delays flowering. We suggest that FT binds to diurnally changing molecular species of PC to promote flowering. FT specifically binds PC in vitro To examine whether FT protein exhibits lipid-binding properties, we performed a lipid ligand screen using membrane-lipid overlay assays. Recombinant and purified His-tagged FT protein was hybridized with a lipid-spotted strip and detected using anti-His antibodies. In this assay a clear and specific binding of His-FT to PC was detected ( Fig. 1a ). The signal was unlikely to be caused by a non-specific association of FT to the lipid by hydrophobic interactions because no binding to any other glycerolipids on the strip was detected. In particular no signals were found for binding to PE, even if PE was spotted at higher concentrations ( Fig. 1b ). This was further confirmed by specific binding of His-FT to PC, but not significantly to PE, purified from Arabidopsis ( Fig. 1c ). Also no binding of His protein (without FT) to the PC spot was detected ( Supplementary Fig. 1 ). We confirmed the binding specificity to PC by liposome protein association assays. As the ratio of PC:PE increased in the liposomes, a stronger binding of FT to the liposomes was observed ( Fig. 1d ). We concluded that FT is a PC-binding protein in vitro . 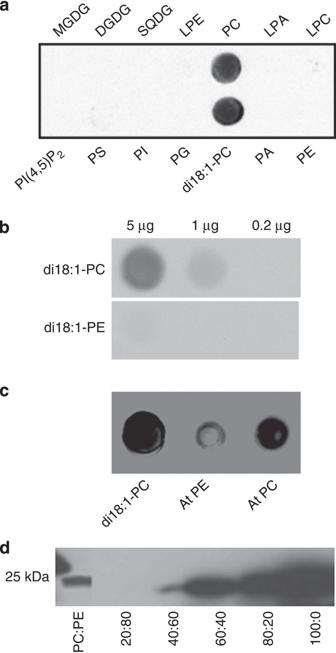Figure 1: FT protein binding to phosphatidylcholine (PC). (a) Membrane-lipid overlay assay with different glycerolipids. A specific binding to PC was observed. Purified, soluble His-tagged FT protein was incubated with a membrane containing different glycerolipid spots as indicated. Lipid-protein binding was visualized with a peroxidase-coupled anti-His antibody and chemiluminescence. A representative membrane of three biological replicates is shown. (b) Comparison of FT binding to PC and PE. Different amounts of di18:1-PC or di18:1-PE were spotted onto the membrane and probed with His-tagged FT protein. (c) FT binding to PC and PE purified from Arabidopsis. Total lipid was extracted from rosette leaves grown in LD, and PC and PE were purified and quantified for spotting on the membrane. (d) Liposome association assay to confirm specific binding of FT to PC. Purified soluble His-tagged FT protein was incubated with liposomes containing different PC:PE ratios. After collecting the liposomes by centrifugation, the portion of FT bound to the liposomes was detected by western blotting using anti-His antibodies. A representative blot of three biological replicates is shown. The left lane shows the position of the protein size marker (25 kDa). Figure 1: FT protein binding to phosphatidylcholine (PC). ( a ) Membrane-lipid overlay assay with different glycerolipids. A specific binding to PC was observed. Purified, soluble His-tagged FT protein was incubated with a membrane containing different glycerolipid spots as indicated. Lipid-protein binding was visualized with a peroxidase-coupled anti-His antibody and chemiluminescence. A representative membrane of three biological replicates is shown. ( b ) Comparison of FT binding to PC and PE. Different amounts of di18:1-PC or di18:1-PE were spotted onto the membrane and probed with His-tagged FT protein. ( c ) FT binding to PC and PE purified from Arabidopsis. Total lipid was extracted from rosette leaves grown in LD, and PC and PE were purified and quantified for spotting on the membrane. ( d ) Liposome association assay to confirm specific binding of FT to PC. Purified soluble His-tagged FT protein was incubated with liposomes containing different PC:PE ratios. After collecting the liposomes by centrifugation, the portion of FT bound to the liposomes was detected by western blotting using anti-His antibodies. A representative blot of three biological replicates is shown. The left lane shows the position of the protein size marker (25 kDa). Full size image PC levels are correlated with flowering time in vivo PC and PE are primary phospholipid constituents of cellular membranes. The contributions of different pathways for PC biosynthesis are still unclear. However, the enzyme CTP:phosphorylethanolamine cytidylyltransferase1 (PECT1) is rate-limiting for PE biosynthesis and thus determines the PC:PE ratio in overall polar glycerolipid composition [13] . While a null mutation of PECT1 in Arabidopsis results in embryonic lethality, the partial suppression of PECT1 activity increases PC levels at the expense of PE, causing a growth retardation of seedlings [13] . We designed a system to alter PC levels in vivo by creating a transgenic plant that harbours pOP::amiPECT1 p35S::GRLhG4 , in which a specific artificial micro RNA designed to target PECT1 mRNA is expressed from the dexamethasone (DEX)-inducible OP promoter [14] , [15] . The obtained lines expressed amiPECT1 even in the absence of DEX and expression of PECT1 was constitutively reduced by about 60% in 9-day-old shoot apical meristems ( Fig. 2a ) and a related increase in PC levels was observed in whole seedlings ( Fig. 2b ). These lines did not show any other visible growth defect, however, continuous treatment with DEX caused growth retardation similar to that observed previously in the leaky mutants of PECT1 ( Supplementary Fig. 2 ; ref. 13 ). Interestingly, the transgenic plants were early flowering, but showed no other growth defect ( Fig. 2c ). In addition, we tested the effects on flowering time of mutations in genes that encode enzymes involved in PC or PE biosynthesis, such as CTP:phosphorylcholine cytidylyltransferase1 (CCT1), CCT2 and phosphorylethanolamine N -methyltransferase 1 (PEAMT1). However, none of these mutations altered flowering time ( Supplementary Fig. 3 ), maybe because as previously reported, mutations in CCT1 or CCT2 do not detectably affect PC levels [16] , and the effect of mutation in PEAMT1 on PC levels was mainly detected in roots [17] . We then examined whether the early-flowering phenotype of amiPECT1 plants was spatially related to FT activity by creating transgenic plants that express amiPECT1 specifically in the phloem companion cells and shoot apical meristems, tissues where FT is present during floral induction. The promoters of SUCROSE TRANSPORTER2 (SUC2) and FD, which are active in the companion cells and shoot meristems respectively, were used to drive amiPECT1 transcription. The pFD::amiPECT1 transgenic lines showed a significantly early-flowering phenotype observed both by leaf number and days to flower ( Fig. 2d ; Supplementary Fig. 4 ), while pSUC2::amiPECT1 transgenic plants flowered at a similar time to wild type. Plants overexpressing PECT1 in the shoot apical meristems were then constructed using a pFD::PECT1 construct and these plants were late flowering compared with the wild type ( Fig. 2e ). We concluded that PC levels at the shoot apical meristems are correlated with flowering time in a dose-dependent manner. 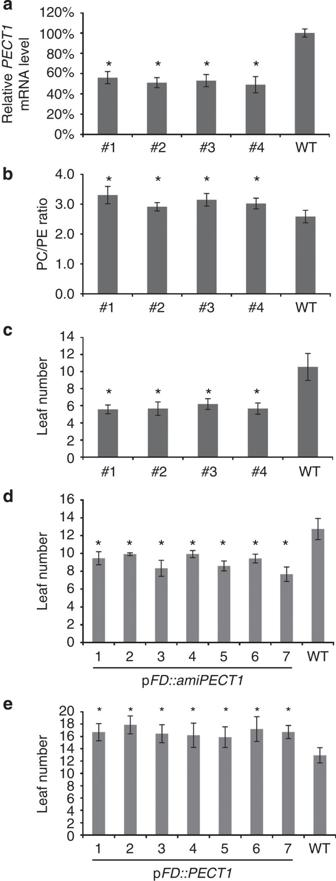Figure 2: Alterations in PC levels affect flowering time. (a–c) Transgenic plant lines that harbourpOP::amiPECT1, 35S::GRLhG4showed constitutively reducedPECT1expression (a), increased PC levels (b) and early flowering (c). (d)pFD::amiPECT1transgenic plants showed a significantly early flowering phenotype. (e)pFD::PECT1 transgenic plants showed late flowering, opposite to the effect observed in (d). Data were averaged by three biological replicates (a,b) and 16 plants (c–e) with standard deviation as error bars. Asterisks show statistical significance (P-value <0.01, Student’st-test). Figure 2: Alterations in PC levels affect flowering time. ( a – c ) Transgenic plant lines that harbour pOP::amiPECT1, 35S::GRLhG4 showed constitutively reduced PECT1 expression ( a ), increased PC levels ( b ) and early flowering ( c ). ( d ) pFD::amiPECT1 transgenic plants showed a significantly early flowering phenotype. ( e ) pFD ::PECT1 transgenic plants showed late flowering, opposite to the effect observed in ( d ). Data were averaged by three biological replicates ( a , b ) and 16 plants ( c – e ) with standard deviation as error bars. Asterisks show statistical significance ( P -value <0.01, Student’s t -test). Full size image The early flowering is related to FT activity The early flowering associated with elevated PC levels at the shoot apex and the in vitro binding of FT to PC suggested that the early flowering could be caused by increased FT signalling. This idea was supported by the higher expression levels of two effectors of FT, AP1 and SOC1 , detected by qRT–PCR (quantitative PCR with reverse transcription) in pFD::amiPECT1 plants compared with wild type ( Fig. 3a,b ). A further test of this hypothesis was to examine whether the elevated PC levels caused by expressing amiPECT1 affect flowering time in the absence of FT . To this end pFD::amiPECT1 was introduced into ft-10 tsf-1 plants that are devoid of FT and its minor functional paralog TWIN SISTER OF FT ( TSF ) ( Supplementary Table 1 ). Introduction of pFD::amiPECT1 into wild-type background accelerated flowering time so that transgenic plants had around 60% of the number of leaves produced by wild type ( Fig. 3c ) at flowering time. However, in ft-10 tsf-1 the early flowering effect was attenuated, so that pFD::amiPECT1 ft-10 tsf-1 plants produced about 80% of the number of leaves of ft-10 tsf-1 plants ( Fig. 3c ) at flowering. Next, to test whether pFD::amiPECT1 can further enhance the early flowering caused by overexpressing FT , pFD::amiPECT1 was introduced into pGAS1::FT ft-10 tsf-1 plants (ref. 18 ). As shown in Fig. 3d , the flowering time was further accelerated and the leaf number was reduced to about 70% of the pGAS1::FT ft-10 tsf-1 plants. We concluded that elevated PC levels in the shoot apex promote flowering mainly through FT. 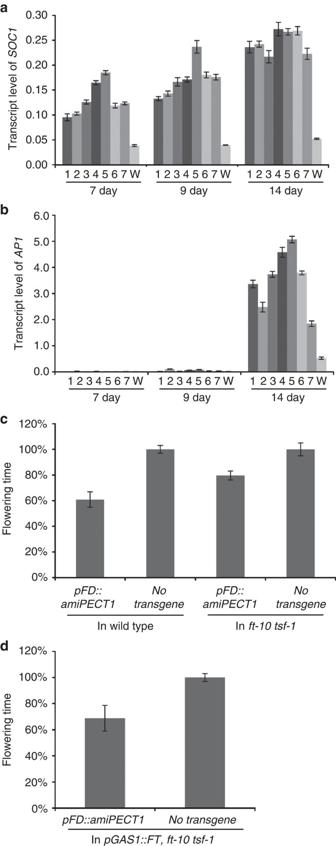Figure 3: Impact of alterations in PC level on the expression of known flowering time control genes. (a,b) Increased expression ofSOC1(a) andAP1(b) inpFD::amiPECT1plants of 7, 9 and 14 days after germination under LD condition. In each time point, seven independent transgenic lines and wild type as a control (indicated as 1–7 and W) were examined with three biological replicates with standard deviation as error bars. (c) Stable expression ofpFD::amiPECT1inft-10 tsf-1plants attenuated the early flowering effect ofpFD::amiPECT1observed in the wild-type background. (d) Stable expression ofpFD::amiPECT1in an FT-overexpressing line (pGAS1::FT, ft-10 tsf-1) further accelerated the flowering time. Data from 16 transgenic plants were averaged with standard deviation as error bars. Y axes in (c,d) are the number of leaves at flowering time relative to the control plants that do not harbor thepFD::amiPECT1transgene. Figure 3: Impact of alterations in PC level on the expression of known flowering time control genes. ( a , b ) Increased expression of SOC1 ( a ) and AP1 ( b ) in pFD::amiPECT1 plants of 7, 9 and 14 days after germination under LD condition. In each time point, seven independent transgenic lines and wild type as a control (indicated as 1–7 and W) were examined with three biological replicates with standard deviation as error bars. ( c ) Stable expression of pFD::amiPECT1 in ft-10 tsf-1 plants attenuated the early flowering effect of pFD::amiPECT1 observed in the wild-type background. ( d ) Stable expression of pFD::amiPECT1 in an FT-overexpressing line ( pGAS1::FT, ft-10 tsf-1 ) further accelerated the flowering time. Data from 16 transgenic plants were averaged with standard deviation as error bars. Y axes in ( c , d ) are the number of leaves at flowering time relative to the control plants that do not harbor the pFD::amiPECT1 transgene. Full size image Specific molecular species of PC oscillate diurnally Given that PC is a major phospholipid in plant membranes, how could a global increase in PC levels stimulate specific FT function in the promotion of flowering? PC as a glycerolipid is characterized by variation in its acyl composition conferring different physical properties. The acyl composition continuously changes according to changing environmental factors such as light, temperature and atmospheric constituents [19] . Moreover, light control of fatty acid synthesis results in a diurnal fluctuation of fatty acid composition in each phospholipid class [20] . We hypothesized that FT might interact with a particular PC molecular species that is dominant at the end of the day when FT accumulates. In this context, we employed a lipidomic profiling approach to monitor diurnal fluctuations of glycerolipid molecular species under short day (SD; 8 h light and 16 h dark) and long day (LD; 16 h light and 8 h dark) in the leaves. Interestingly, PC molecular species showed clear diurnal changes whereas there was no such profile for PE ( Fig. 4a–d ). During the light period, PC species containing less unsaturated fatty acids (36:4, 36:3, 36:2, 36:1 and 34:1) were predominant, while in the dark period those containing linolenic acid (36:6 and 36:5) were increased. This profile was in agreement with a previous report on diurnal oscillation of total and PC-bound fatty acids [20] , suggesting that the molecular species of PC, but not of PE, were under diurnal regulation. We therefore examined binding of FT to PC with different acyl groups. The lipid-protein overlay assay showed that binding of FT to di18:3-PC (36:6), a predominant molecular species in the dark period, was significantly lower compared with the other more saturated PC species ( Fig. 4e and Supplementary Fig. 5 ). The weaker binding of FT to di18:3-PC was confirmed at different concentrations ( Fig. 4f ). This suggests that PC molecular species that are preferentially bound by FT are scarce during the dark period, and therefore less FT is bound to PC at these times. To further examine if an increase in 18:3-containing PC species delays flowering, we tested the flowering time of the transgenic line CS8035, which overexpresses FATTY ACID DESATURASE3 ( FAD3 ) catalysing the desaturation of 18:2 in PC to 18:3, leading to an increase in 18:3 in PC (ref. 21 ). As expected, our data indicated that flowering time of CS8035 was significantly delayed compared with the wild type under LD conditions ( Fig. 4g ), suggesting that the presence of a high proportion of 18:3-PC delays flowering. Taken together, these data support a model whereby FT preferentially interacts with PC species that are predominant in the light period to promote flowering at the correct time. 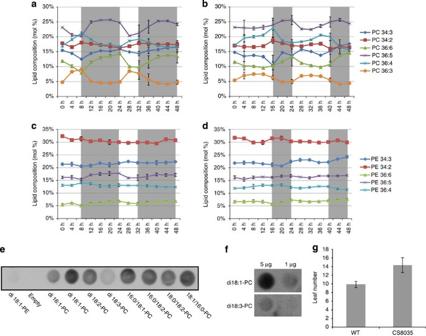Figure 4: Diurnal oscillation of PC molecular species and selective binding of FT to PC species dominant at daytime. (a–d) Lipidomic profiling of PC and PE species under SD (aandc, respectively) or LD (bandd, respectively). Seedlings were germinated and grown for 2 weeks under SD, shifted to either LD or SD and time-course dependent harvesting started 24 h after shifting the plants. Data show averages and standard deviation of four biological replicates. Grey boxes indicate the dark period. (e) Membrane-lipid overlay assay of different PC molecular species with His-tagged FT protein. (f) Weaker binding of FT to di18:3-PC at different concentration of lipids. The photos of the membranes after binding in (e) and (f) are representative of three replicates. (g) Leaf number at flowering time of CS8035 plants under LD. Data were averaged by 16 plants with standard deviation as error bars. Figure 4: Diurnal oscillation of PC molecular species and selective binding of FT to PC species dominant at daytime. ( a – d ) Lipidomic profiling of PC and PE species under SD ( a and c , respectively) or LD ( b and d , respectively). Seedlings were germinated and grown for 2 weeks under SD, shifted to either LD or SD and time-course dependent harvesting started 24 h after shifting the plants. Data show averages and standard deviation of four biological replicates. Grey boxes indicate the dark period. ( e ) Membrane-lipid overlay assay of different PC molecular species with His-tagged FT protein. ( f ) Weaker binding of FT to di18:3-PC at different concentration of lipids. The photos of the membranes after binding in ( e ) and ( f ) are representative of three replicates. ( g ) Leaf number at flowering time of CS8035 plants under LD. Data were averaged by 16 plants with standard deviation as error bars. Full size image According to the FAC model, the final destination of FT is the nuclei of cells in the shoot apical meristem [9] . Since PC is synthesized at the ER and is a component of the nuclear membrane as well, it is possible that PC at the nuclear membrane attracts free FT from the cytosol for efficient import into the nucleus. Alternatively, PC-containing vesicles could be a part of FAC, mediating trafficking of FT. Furthermore, FT homologues might also bind PC or other phospholipids. For example, TERMINAL FLOWER1 (TFL1) is highly similar to FT in sequence and three-dimensional structure, yet they have opposite function in controlling flowering [22] . This might explain why pFD::amiPECT in ft-10 tsf-1 plants still weakly accelerated flowering time ( Fig. 3c ). However, monitoring precise PC distribution at the subcellular level awaits further development of techniques for lipid analysis at this resolution. The clear FT binding to PC, the gene effector expression analysis as well as the genetic data showing altered flowering times suggest that at least one PC species interacts with FT and enhances its activity. Moreover, this lipid binding is likely important for FT function, as several loss-of-function mutants of FT ( ft-3 , ft-4 and ft-6 ; ref. 22 ) carry point mutations within the ligand-binding pocket. Nevertheless, the genetic approach to alter PC levels may also affect the production of PC metabolites, such as diacylglycerol, phosphatidic acid (PA) or lysoPC. Moreover, the proportion of PC with regard to other lipids might be crucial for the binding of FT to vesicles. In conclusion, our study suggests that the florigen FT binds to diurnally changing PC molecular species to promote flowering. Plant material The T-DNA line CS8035 (overexpressing FAD3 ) was obtained from TAIR, a double mutant ft-10 tsf-1 and a transgenic line pGAS1::FT ft-10 tsf-1 were previously described [18] . pFD::amiPECT1, ft-10 tsf-1 and pFD::amiPECT1, pGAS1::FT ft-10 tsf-1 were created by crossing pFD::amiPECT plant (line no. 2) with ft-10 tsf-1 or pGAS1::FT ft-10 tsf-1 , respectively. Detection of the transgenes pFD::amiPECT1 and pGAS1::FT was performed by PCR using the primer pairs YN1276 and YN1277, or YN1279 and YN1280, respectively ( Supplementary Table 2 ). Growth condition and observation Flowering time was observed under long day (LD; 16 h light and 8 h dark) or short day (SD; 8 h light and 16 h dark) with the light intensity of 150 μmol m −2 s −1 and 21 °C. Harvesting of seedlings for lipidomic profiling during a time course experiment was performed as previously described [2] . Expression and purification of His-tagged FT protein The protein coding sequence of FT was amplified with primers KK176 and KK177, and cloned into the Sph I/ Kpn I sites of the pQE30 expression vector (Qiagen) to obtain pYN1041 (pQE30-His-FT). The plasmid pYN1041 was transformed into the Escherichia coli strain AD16 (ref. 23 ) and cultured in M9 media. Protein expression was induced at an OD 600 of about 0.4 by adding IPTG (isopropyl β-D-1-thiogalactopyranoside) to the M9 culture growing at 37 °C, then the temperature was shifted to 23 °C and the cells grown overnight to express His-FT in a soluble form. The expressed protein was batch-purified with Ni-NTA resin (Qiagen) according to the manufacturer's instructions. Protein lipid overlay assay Membrane strips used for the FT-lipid overlay assay were prepared by spotting approximately 5 μg of commercially available lipids onto Hybond P ECL+ (Amersham Biosciences). Lipid standards were purchased from Avanti Polar Lipids or Sigma. The hybridization was performed essentially according to Awai et al. [24] except that a horseradish peroxidase–coupled antibody (sc-8036, Santa Cruz Biotechnology, TX) against histidine was used at a 1:10,000 dilution, and the protein bound to the lipid spot was detected by chemiluminescence substrates (SuperSignal West Pico Maximum Sensitivity Substrate, Thermo Scientific, Rockford, IL) and image analyser (LAS4000, GE healthcare). The lipid molecular species used for the FT protein binding to different glycerolipids ( Fig. 1a ) were: PA, 1,2-dioleoyl phosphatidic acid; PC, PC purified from egg yolk; di18:1-PC, 1,2-dioleoyl phosphatidylcholine; PE, 1,2-dioleoyl phosphatidylethanolamine; PG, 1,2-dioleoyl phosphatidylglycerol; PI and PS, phosphatidylinositol and phosphatidylserine purified from soybean; MGDG and DGDG, monogalactosyldiacylglycerol and digalactosyldiacylglycerol purified from whole-wheat flour and PI(4,5)P 2 , 1,2-dipalmitoyl phosphatidylinositol 4,5-bisphosphate. The PC molecular species employed for the lipid overlay assay shown in Fig. 1b,c ; Fig. 4e and f (di16:1-PC, di18:2-PC, di18:3-PC, 16:0/18:1-PC, 16:0/18:2-PC, 18:0/18:2-PC, 18:1/16:0-PC; sn- 1/ sn- 2) were obtained from Avanti Polar Lipids. AtPC and AtPE were PC and PE purified from Arabidopsis leaves, respectively. A total of 5 μg of lipid were applied onto each spot. Signal intensity of each spot was quantified by image analyser (LAS4000, GE healthcare). Liposome association assay The liposome association assay was performed as described [25] , [26] . Lipids were dried and incubated in Tris buffered saline (TBS) (50 mM Tris-HCl, pH 7.0, 0.1 M NaCl) at 37 °C for 1 h. The liposomes were formed by vigorous vortexing (5 min), pelleted by centrifugation at 20,000 × g for 10 min at 4 °C, and washed twice with ice-cold TBS. Purified His-FT was added to the liposomes to a final 100 μl volume, and the mixture was incubated at 30 °C for 30 min. After incubation, liposomes were pelleted again by centrifugation at 20,000 × g and washed twice with ice-cold TBS. The pellets were analysed by SDS–polyacrylamide gel electrophoresis and blotted onto nitrocellulose membrane (Bio-Rad, Hercules, CA) for protein gel blot analysis. His-FT was immunodetected by a monoclonal antibody against penta-His (H1029, Sigma-Aldrich; dilution 1:1,000) and horseradish peroxidase–coupled anti-mouse IgG (A3682, Sigma-Aldrich; dilution 1:10,000) with the West Pico chemiluminescence detection kit (Thermo Scientific, Rockford, IL) and signal intensity of each spot was quantified by image analyser (LAS4000, GE healthcare). An uncropped scan of a representative result is shown in Supplementary Fig. 6 . Construction of transgenic lines The amiRNA targeting PECT1 (At2g38670) was designed with the WMD2 software and following the instructions available at the web site: http://wmd2.weigelworld.org/cgi-bin/mirnatools.pl . miRNA (ACCCCGTATTCTCTACCAATA) and miRNA* (TATTGGTACAGAATACGGGTT) were cloned by PCR into the Arabidopsis precursor MIR319a included in the vector pRS300. The amiRNA precursor fragment was then amplified by using primers containing Gateway sites (F206 and F207) and subcloned by RB reaction in a pDONR207 vector (Invitrogen). LR recombination was performed to transfer the amiRNA precursor fragment to the binary vectors pSUC2 ::GW [2] and pFD ::GW to generate the pSUC2 ::amiPECT1 and pFD ::amiPECT1 constructs, respectively. pFD ::GW was generated from the vector pLEELA [27] in which the 2 × 35S promoter was replaced at the Asc I/ Xho I restriction sites by 2.8 Kbs of the FD promoter. The CDS of PECT1 was amplified with the primers PECT1_gw_F and PECT1_gw_R and cloned by LR recombination into pFD ::GW to generate pFD ::PECT1. Plants were transformed with Agrobacterium tumefaciens strain GV3101 pMP90 RK by floral dipping [28] . The primer sequences used for cloning are listed in the Supplementary Table 2 . qRT–PCR analysis of gene expression Total RNA was extracted using the RNAeasy kit (Qiagen) and treated with DNaseI (Ambion). cDNA synthesis was performed with SuperScript II (Invitrogen) from 1–3 μg of DNA free RNA and diluted to a final volume of 200 μl with water. A total of 3 μl of diluted cDNA were used for each quantitative RT–PCR (qRT-PCR) reaction. qRT–PCR reactions were prepared using the iQ SYBR Green supermix (Bio-Rad) and performed in a LightCycler 480 thermal cycler (Roche). PEX4 (At5g25760) was used as a housekeeping gene to normalize the expression of the genes investigated. The primer sequences used for qRT–PCR experiments are listed in the Supplementary Table 2 . Total lipid extraction Frozen tissue was immersed in boiling water for 20 min, then the water was replaced by one part of chloroform: methanol=1:2 (vol/vol). The solvent was collected and the same volume of chloroform: methanol=2:1 (vol/vol) added to the tissue for the second extraction. The two extracts were combined and one part of chloroform and 0.75 part of NaCl solution (0.5%) were added, mixed and centrifuged to separate the organic phase from the aqueous phase. The isolated organic phase was dried under a nitrogen stream and lipids were dissolved in chloroform: methanol=2:1 and stored at −20 °C. Lipidomic profiling Lipid analysis in Fig. 2b was performed essentially as described previously [29] . Briefly, major polar glycerolipids (MGDG, DGDG, SQDG, PC, PE, PG and PI) were separated on two-dimensional TLC by the solvent system of chloroform:methanol: 7N ammonia solution=120:80:8 (vol/vol/vol) for the first dimension and chloroform:methanol:acetic acid:water=170:20:15:3 (vol/vol/vol/vol) for the second dimension. Each spot was scraped off, lipid re-extracted and methylesterified to fatty acid methyl esters, which were quantified by gas chromatography (GC-2010; Shimadzu, Kyoto, Japan) with a capillary column (ULBON HR-SS-10, Shinwa Chemical Industries, Kyoto, Japan). For glycerolipid quantification in Fig. 4a–d , an aliquot of the lipid sample was diluted in methanol:chloroform:300 mM ammonium acetate (665:300:35) [30] . Two internal phospholipid standards each were added for PC, PE, PG, PA and PS (Avanti Polar Lipids) to the samples [30] . The lipid standards MGDG, DGDG, SQDG and PI (Larodan) were hydrogenated before addition to the sample [31] . The samples were supplied to a Q-TOF (quadrupole time-of-flight) mass spectrometer (Q-TOF 6530; Agilent) in chloroform/methanol/ 300 mM ammonium acetate (300:665:35; ref. 30 ) at a flow rate of 1 μl min −1 with a nanospray ion source (HPLC Chip/MS 1200 with infusion chip; Agilent). After ionization in the positive mode with a fragmentor voltage of 270 V, ammonium or proton adducts [32] were selected in the quadrupole and fragmented in the collision cell [30] . After correction for isotopic overlap, lipid molecular species were quantified [32] . How to cite this article: Nakamura, Y. et al. Arabidopsis florigen FT binds to diurnally oscillating phospholipids that accelerate flowering. Nat. Commun. 5:3553 doi: 10.1038/ncomms4553 (2014).